mTORC1-independent Raptor prevents hepatic steatosis by stabilizing PHLPP2 Mechanistic target of rapamycin complex 1 (mTORC1), defined by the presence of Raptor, is an evolutionarily conserved and nutrient-sensitive regulator of cellular growth and other metabolic processes. To date, all known functions of Raptor involve its scaffolding mTOR kinase with substrate. Here we report that mTORC1-independent (‘free’) Raptor negatively regulates hepatic Akt activity and lipogenesis. Free Raptor levels in liver decline with age and in obesity; restoration of free Raptor levels reduces liver triglyceride content, through reduced β-TrCP-mediated degradation of the Akt phosphatase, PHLPP2. Commensurately, forced PHLPP2 expression ameliorates hepatic steatosis in diet-induced obese mice. These data suggest that the balance of free and mTORC1-associated Raptor governs hepatic lipid accumulation, and uncover the potentially therapeutic role of PHLPP2 activators in non-alcoholic fatty liver disease. Obesity-induced metabolic dysfunction manifests as multiple chronic medical conditions, including type 2 diabetes (T2D) and non-alcoholic fatty liver disease (NAFLD) [1] . NAFLD contributes to the overall cardiovascular risk of obesity [2] , but is also the most common chronic liver disease, predisposing to cirrhosis and hepatocellular carcinoma [3] . Ageing and obesity are well-established risk factors for NAFLD [4] , but the molecular mechanism underlying this risk is poorly defined, precluding specific pharmacologic strategies to target excess hepatic triglycerides. The evolutionarily conserved mechanistic target of rapamycin (mTOR) is a phosphatidylinositol 3-kinase (PI3K)-like serine/threonine kinase that regulates cell growth in response to nutrient signals [5] , as well as a recently discovered regulatory role in lipid homoeostasis. Mice with liver-specific deletion of the mTOR complex 1 (mTORC1)-defining subunit Raptor ( L-Raptor ) show reduced SREBP (sterol regulatory element (SRE)-binding protein)-1c-dependent de novo lipogenesis (DNL) and are thus protected from fatty liver [6] . Inhibition of mTOR/Raptor interaction with the allosteric mTORC1 inhibitor rapamycin similarly blocks insulin-dependent SREBP1c activation in primary rat hepatocytes and liver [7] , [8] , [9] . Consistently, SREs are highly enriched in promoters of rapamycin-sensitive genes [10] , leading to the conclusion that mTORC1 is required for the lipogenic actions of insulin. Surprisingly, mice with liver-specific deletion of Tsc1 ( L-Tsc1 ), the endogenous inhibitor of mTORC1, are also spared from both age- and diet-induced hepatic steatosis [9] . The molecular mechanism underlying this apparent contradictory result was discovered to be feedback inhibition preventing normal activation of the serine–threonine kinase Akt [9] , which then interferes with SREBP1c function via modulation of Insig2a expression [11] , [12] . Akt is a critical molecular node in insulin signal transduction to both gluconeogenic and lipogenic liver pathways [9] , [13] , [14] . As such, mice lacking both hepatic Akt isoforms show marked defects in both insulin-mediated metabolic processes in liver—glucose intolerance [15] , primarily but not exclusively due to loss of its inhibitory action on the gluconeogenic transcription factor FoxO1 (ref. 16 ), as well as a similar reduction in feeding-induced Srebp1c expression as mice lacking hepatic insulin receptor [17] . Collectively, these results point to Akt activity as a key regulator of insulin action in liver, and suggest that it affects DNL via both mTORC1-dependent and -independent mechanisms. Akt is primarily regulated by post-transcriptional means—insulin stimulation of PI3K induces membrane localization, unmasking Thr308 for phosphorylation by PDK1, which then triggers mTORC2 (mTOR complex 2)-mediated phosphorylation at Ser473 (refs 18 , 19 ). While the necessity for both Thr308/Ser473 phosphorylation events in physiologic Akt activation is well-established [20] , [21] , [22] , mechanisms accounting for termination or negative regulation of Akt signalling are far less understood. Our lab has shown that altered mTORC1 complex stability is associated with increased Akt activity [23] —although this phenotype may be attributed to circumvention of normal nutrient-regulated mechanisms of mTORC1 catalytic activity and feedback regulation of Akt [24] , we hypothesized that mTORC1 stability has an additional, indirect role to terminate the Akt signal. Herein we show that Raptor exists in both the mTORC1-bound and -independent (‘free’) state in liver of young, healthy mice, but that free Raptor levels decline markedly in ageing and obesity, coupled with increased Akt activity and hepatic triglyceride. Moderate hepatic Raptor overexpression to correct the free Raptor deficit reversed Akt hyperactivity, decreasing DNL and hepatic triglyceride accumulation by increasing protein stability of the recently identified Akt Ser473 phosphatase Pleckstrin homology (PH) domain leucine-rich repeat protein phosphatase 2 (PHLPP2) [25] , [26] . Raptor overexpression prevents aging- or high-fat diet (HFD)-mediated reductions in PHLPP2 levels, without adversely affecting either mTORC1/2 activity or whole-body glucose homoeostasis. Consistently, mild hepatic PHLPP2 overexpression reduced lipogenic gene expression and obesity-induced triglyceride accumulation, without affecting glucose tolerance. These data suggests an important modulatory action of the balance in free and mTORC1-bound Raptor in the bifurcation model of hepatic insulin action, as well as point to PHLPP2 as a novel therapeutic target for NAFLD. Free Raptor levels decline in aged and obese liver mTORC1 complexes are affected by hormonal signals and oxidative stress [24] , [27] , likely through direct effects on mTORC1 subunits, and modulated by other upstream signals, such as IPMK and Notch [23] , [28] . These data suggest that the mTOR/Raptor interaction is fluid. As liver-specific Raptor ( L-Raptor ) knockout mice show aging-dependent defects in ketogenesis [29] and obesity-dependent reductions in lipogenesis [6] , we hypothesized that mTORC1 component interaction may be altered in these pathophysiologic processes. We performed size-exclusion chromatography to fractionate detergent-free liver lysate from young mice, and in parallel, older or leptin-deficient ( ob/ob ) obese mice. In all three groups of mice, mTOR and GβL eluted in high-molecular weight ( ∼ 800 kDa) fractions ( Fig. 1a,b ), consistent with mTORC1 complex dimers [27] , [30] , [31] . Raptor was also found mostly in high-molecular weight fractions in older or obese mice, but livers from young mice showed a surprising amount of ‘free’ ( ∼ 150 kDa) Raptor ( Fig. 1a,b ). We next sought confirmation of this finding using alternative biochemical methods. We exposed liver lysate to a cell-permeable, non-cleavable chemical cross-linker to trap native mTORC1 complexes, and again observed a marked decrease of free Raptor with aging or obesity, without change in other mTORC1/2 component distribution ( Fig. 1c,d and Supplementary Fig. 1a–c ). As total levels of mTOR and Raptor did not substantially change, we hypothesized that altered free Raptor reflected greater mTOR–Raptor association in aging or obesity. To test this, we exposed liver lysate to a cleavable cross-linker to ensure complete recovery of mTORC1 components. As predicted, whereas the interaction between mTOR and GβL was unchanged, mTOR–Raptor association was markedly increased in ob/ob mice ( Supplementary Fig. 1d ). Consistently, performing anti-mTOR immunoprecipitation using CHAPS detergent to sustain the mTOR–Raptor interaction in the absence of cross-linker [24] , we found greater bound Raptor in ob/ob mice ( Supplementary Fig. 1e ). 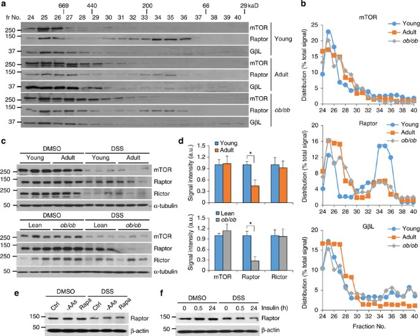Figure 1: Free Raptor levels decline in aged and obese liver. (a,b) Western blot from livers of young (8-week-old), adult (24-week-old) andob/ob(8-week-old) male mice, following size-exclusion chromatography (a) and quantification of signal per fraction (b), normalized to total protein. (c,d) Western blot from livers of young, adult andob/obmale mice, cross-linked with disuccinimidyl suberate (DSS) (c) and quantification of free Raptor signal (d), as a percentage of control (dimethylsulphoxide (DMSO)-treated liver lysate). (e,f) Western blot from hepatocytes deprived of amino acids or treated with rapamycin (e), or insulin (f), before disuccinimidyl suberate crosslinking. *P<0.05 as compared with the indicated control by two-way analysis of variance. All data are shown as the means±s.e.m. All blots are representative of three independent experiments, and samples within each group chosen randomly. Figure 1: Free Raptor levels decline in aged and obese liver. ( a , b ) Western blot from livers of young (8-week-old), adult (24-week-old) and ob/ob (8-week-old) male mice, following size-exclusion chromatography ( a ) and quantification of signal per fraction ( b ), normalized to total protein. ( c , d ) Western blot from livers of young, adult and ob/ob male mice, cross-linked with disuccinimidyl suberate (DSS) ( c ) and quantification of free Raptor signal ( d ), as a percentage of control (dimethylsulphoxide (DMSO)-treated liver lysate). ( e , f ) Western blot from hepatocytes deprived of amino acids or treated with rapamycin ( e ), or insulin ( f ), before disuccinimidyl suberate crosslinking. * P <0.05 as compared with the indicated control by two-way analysis of variance. All data are shown as the means±s.e.m. All blots are representative of three independent experiments, and samples within each group chosen randomly. Full size image Although the disappearance of free Raptor in the liver from aging or obese mice was consistent across multiple experimental platforms, we remained skeptical, as various in vitro manipulations have been shown to affect biochemical recovery of mTORC1 complexes without true impact on mTOR–Raptor binding [24] , [32] . For instance, transient amino acid deprivation increases, while rapamycin treatment decreases immunoprecipitation efficiency of Raptor ( Supplementary Fig. 1f ), but neither stimulus altered free Raptor levels ( Fig. 1e ). This suggests that our observation of free Raptor in young liver is likely through a novel mechanism, and that nutrient and/or hormonal signals prompts a true change in Raptor–mTOR association. We investigated this possibility in vitro , to dissociate the various components of obesity and found that while transient/chronic hyperglycaemia or brief insulin exposure were ineffectual, prolonged high-dose insulin treatment to induce insulin resistance [33] reduced free Raptor ( Fig. 1f and Supplementary Fig. 1g ). Thus, hepatocyte insulin resistance is sufficient to reduce free Raptor levels. Rescue of free Raptor levels prevents hepatic steatosis We next hypothesized that loss of free Raptor in the insulin-resistant state, beyond the above correlation, may be causative to aging/obesity-induced metabolic dysfunction, which in liver manifests as excessive triglyceride content, or hepatic steatosis. To test this, we transduced adult mice with adenovirus encoding Raptor (Ad-Raptor) or green fluorescent protein (GFP) control (Ad-GFP) to acutely increase the hepatic Raptor/mTOR ratio, and increase free Raptor levels ( Fig. 2a ). As a further internal control, we transduced young mice, which have ‘normal’ free Raptor levels ( Supplementary Fig. 2a ). While we observed no benefit in young mice, suggestive of a threshold effect of free Raptor, aging-induced hepatic triglyceride accumulation was blocked by Ad-Raptor delivery ( Fig. 2b ). To push the hypothesis further, we repeated the experiment in aged (12-month-old) or diet-induced obese (DIO) mice, which have further elevations in hepatic triglyceride as compared with young or adult mice ( Supplementary Fig. 2b ). Remarkably, acute increase in free Raptor levels reduced liver triglyceride and liver weight in both aged ( Fig. 2c and Supplementary Fig. 2c ) and DIO mice ( Fig. 2d and Supplementary Fig. 2d ), proving that the observed free Raptor deficit in these states has biological consequence, as replacement can ameliorate aging/obesity-induced hepatic steatosis. 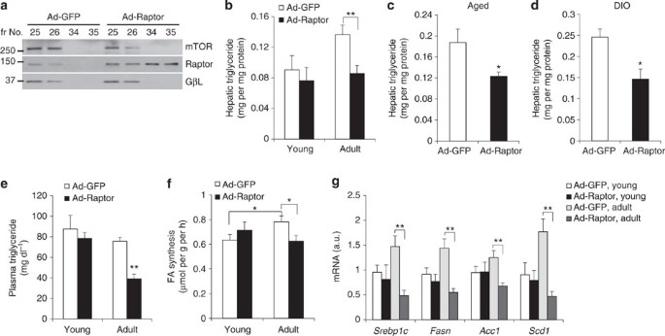Figure 2: Rescue of free Raptor prevents aging- and obesity-dependent hepatic steatosis. (a) Western blot from livers of adult Ad-GFP and Ad-Raptor male mice, following size-exclusion chromatography. Fractions 24 and 25 correspond to mTORC1-associated (∼800 kDa) Raptor, while 34 and 35 to free (∼150 kDa) Raptor. (b–d) Hepatic triglyceride (TG) in young or adult (n=6/group) (b), aged (10- to 12-month-old) (n=7 per group) (c), or DIO (n=5 per group) (d) Ad-GFP and Ad-Raptor male mice. (e–g) Plasma TG (e), hepatic fatty acid synthesis (f) and lipogenic gene expression (g) in young or adult, Ad-GFP and Ad-Raptor mice, killed after a 16 h fast followed by 4 h refeeding (n=6 per group). *P<0.05, **P<0.01 as compared with the indicated control by two-way analysis of variance. All data are shown as the means±s.e.m. All blots are representative of three independent experiments, and samples within each group chosen randomly. Figure 2: Rescue of free Raptor prevents aging- and obesity-dependent hepatic steatosis. ( a ) Western blot from livers of adult Ad-GFP and Ad-Raptor male mice, following size-exclusion chromatography. Fractions 24 and 25 correspond to mTORC1-associated ( ∼ 800 kDa) Raptor, while 34 and 35 to free ( ∼ 150 kDa) Raptor. ( b – d ) Hepatic triglyceride (TG) in young or adult ( n =6/group) ( b ), aged (10- to 12-month-old) ( n =7 per group) ( c ), or DIO ( n =5 per group) ( d ) Ad-GFP and Ad-Raptor male mice. ( e – g ) Plasma TG ( e ), hepatic fatty acid synthesis ( f ) and lipogenic gene expression ( g ) in young or adult, Ad-GFP and Ad-Raptor mice, killed after a 16 h fast followed by 4 h refeeding ( n =6 per group). * P <0.05, ** P <0.01 as compared with the indicated control by two-way analysis of variance. All data are shown as the means±s.e.m. All blots are representative of three independent experiments, and samples within each group chosen randomly. Full size image Given the known hepatocyte tropism of adenovirus [34] , we hypothesized that free Raptor protects from steatosis through a cell–autonomous mechanism, consistent with unchanged body weight, adiposity and plasma fatty acids in Ad-Raptor mice ( Supplementary Fig. 3a–c ). Liver Acox and Cpt1a gene expression and plasma ketone levels were unchanged ( Supplementary Fig. 3d,e ), indicative of normal β-oxidation/ketogenesis. Plasma triglyceride was lower in Ad-Raptor mice ( Fig. 2e ), implying no increase in hepatic triglyceride secretion as very-low-density lipoprotein. Finally, to test DNL, we injected 3 H 2 O into Ad-Raptor and control mice, and measured incorporation of label into newly synthesized hepatic fatty acid. We found that adult mice had higher rates of lipogenesis than young mice, but this was reversed by correcting the aging-related free Raptor defect ( Fig. 2f ). Consistently, we observed reduced expression of Srebp1c , the master regulator of lipogenesis, as well as its transcriptional targets in Ad-Raptor-transduced liver ( Fig. 2g ) and primary hepatocytes ( Supplementary Fig. 3f ). Free Raptor reduces Akt-mediated lipogenesis We next investigated the molecular mechanism underlying free Raptor-mediated reduced lipogenesis. Data from rapamycin-treated hepatocytes and from L-Raptor mice has proven that mTORC1 activity is necessary for normal hepatic Srebp1c function [6] , [8] . If Raptor overexpression reduces mTORC1 catalytic function in liver, similar to in vitro effects observed in HEK293 cells [24] , we would expect impaired Srebp1c-dependent lipogenesis. Ad-Raptor-transduced liver, however, showed normal fasted or refed mTORC1 kinase activity on recombinant 4E-BP1, phosphorylation of canonical mTORC1 targets and hepatic protein content ( Supplementary Fig. 4a–c ), in stark contrast with the phenotype of L-Raptor mice [29] . Consistently, mTORC1-dependent negative feedback on insulin signalling through IRS1 phosphorylation was unchanged ( Supplementary Fig. 4d ). We next tested an alternative hypothesis whereby the addition of excess Raptor could ‘steal’ shared mTOR components from mTORC2, and recapitulate the lower hepatic triglyceride observed in L-Rictor mice [21] , but we observed normal mTOR interaction with Rictor and the shared mTORC1/2 component, GβL ( Supplementary Fig. 4e ). In addition, Ad-Raptor mice showed normal p-Akt Thr450 and PKCα levels ( Supplementary Fig. 4f,g ), which are phosphorylated and stabilized by mTORC2 (refs 35 , 36 ). Interestingly, we did find that phosphorylation of Akt at Ser473, another known mTORC2 substrate, was increased by aging in Ad-GFP, but not Ad-Raptor mice ( Fig. 3a ). PI3K/PDK1-mediated phosphorylation at Thr308 was unaffected ( Fig. 3b ), but we predicted that decreased Akt Ser473 phosphorylation in Ad-Raptor mice would be sufficient to reduce Akt kinase activity [37] . Indeed, GSK3β Ser9 ( Supplementary Fig. 5a ) and general Akt substrate phosphorylation ( Supplementary Fig. 5b ) was lower, as was immunoprecipitated Akt kinase activity on recombinant GSK3β ( Fig. 3c ). In addition, reduced Akt activity in Ad-Raptor livers led to a twofold increase in hepatic Insig2a expression ( Supplementary Fig. 5c ), supporting the conclusion that free Raptor regulates Srebp1c-mediated lipogenesis via an Akt-regulated but mTORC1-independent pathway [9] . 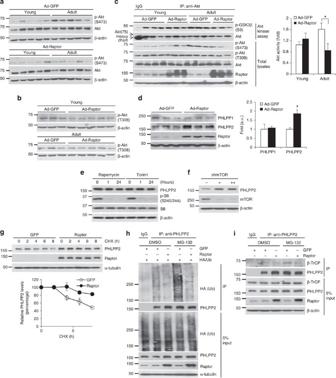Figure 3: Free Raptor reduces Akt hyperactivity by stabilizing PHLPP2. (a,b) Western blots from livers of young or adult Ad-GFP and Ad-Raptor mice killed after a 16 h fast followed by 4 h refeeding. (c) Akt activity on recombinant GSK3β peptide, normalized to immunoprecipitated Akt levels. (d) Western blot from liver of adult Ad-GFP and Ad-Raptor mice killed after a 16 h fast followed by 4 h refeeding, normalized to β-actin. (e) Western blot from Hepa1c1c7 cells treated with Rapamycin (20 nM) or Torin1 (250 nM). (f) Western blot from primary hepatocytes transduced with Ad-shControl or Ad-shmTOR. (g) Western blot of cycloheximide (CHX, 50 mg ml−1)-treated primary hepatocytes transduced with GFP or Raptor adenovirus. Quantification of PHLPP2, normalized to β-actin, relative to time 0 as 100%. (h,i) Western blot of Raptor (or GFP control)-transduced and/or HA/Ub-transfected primary hepatocytes following immunoprecipitation with anti-PHLPP2, with or without MG-132. *P<0.05 as compared with the indicated control by two-way analysis of variance. All blots are representative of three independent experiments, and samples within each group chosen randomly. Figure 3: Free Raptor reduces Akt hyperactivity by stabilizing PHLPP2. ( a , b ) Western blots from livers of young or adult Ad-GFP and Ad-Raptor mice killed after a 16 h fast followed by 4 h refeeding. ( c ) Akt activity on recombinant GSK3β peptide, normalized to immunoprecipitated Akt levels. ( d ) Western blot from liver of adult Ad-GFP and Ad-Raptor mice killed after a 16 h fast followed by 4 h refeeding, normalized to β-actin. ( e ) Western blot from Hepa1c1c7 cells treated with Rapamycin (20 nM) or Torin1 (250 nM). ( f ) Western blot from primary hepatocytes transduced with Ad-shControl or Ad-shmTOR. ( g ) Western blot of cycloheximide (CHX, 50 mg ml −1 )-treated primary hepatocytes transduced with GFP or Raptor adenovirus. Quantification of PHLPP2, normalized to β-actin, relative to time 0 as 100%. ( h , i ) Western blot of Raptor (or GFP control)-transduced and/or HA/Ub-transfected primary hepatocytes following immunoprecipitation with anti-PHLPP2, with or without MG-132. * P <0.05 as compared with the indicated control by two-way analysis of variance. All blots are representative of three independent experiments, and samples within each group chosen randomly. Full size image Raptor increases PHLPP2 levels to terminate Akt signalling Akt Ser473 phosphorylation was not altered in extra-hepatic tissues of Ad-Raptor mice ( Supplementary Fig. 5d ), suggesting a cell-autonomous effect of free Raptor on Akt activity, as opposed to a whole-body change in insulin sensitivity, consistent with normal plasma insulin levels ( Supplementary Fig. 5e ). These data prompted the hypothesis that Akt Ser473 dephosphorylation was increased in Ad-Raptor mice. PHLPPs, encoded by Phlpp1 , with two splice variants (PHLPP1α and PHLPP1β), and Phlpp2, have recently been shown to dephosphorylate Akt Ser473 to terminate insulin/growth factor action [25] , [26] . PHLPP1β and PHLPP2 are expressed in liver ( Supplementary Fig. 6a ), but Raptor overexpression selectively increased PHLPP2 ( Fig. 3d ). PHLPP2 levels were unaffected by mTOR inhibitors ( Fig. 3e and Supplementary Fig. 6b ) or increased mTORC1 activity in Tsc2 knockout ( Tsc2 −/− ) mouse embryonic fibroblasts ( Supplementary Fig. 6c ), but are markedly lower in livers of adult or HFD-fed L-Raptor mice ( Supplementary Fig. 6d,e ) and in shRaptor-transduced primary hepatocytes ( Supplementary Fig. 6f ). Conversely, acute mTOR knockdown to increase the Raptor/mTOR ratio, and thus free Raptor levels, increased hepatocyte PHLPP2 ( Fig. 3f ). In summary, these data prove that free Raptor, but not mTORC1/2 activity, regulates PHLPP2. Interestingly, Raptor overexpression did not increase Phlpp2 mRNA in liver or primary hepatocytes ( Supplementary Fig. 6g,h ), even as it induced protein levels of both basal and exogenous PHLPP2 ( Supplementary Fig. 6i ), suggesting an impact of free Raptor on PHLPP2 stability. Consistent with this hypothesis, Raptor overexpression maintained PHLPP2 levels in the face of cycloheximide treatment ( Fig. 3g ), likely due to reduced ubiquitin-mediated proteosomal degradation ( Fig. 3h ). β-TrCP (beta-transducin repeat-containing protein), the E3 ligase/substrate recognition subunit of the SCF (Skp1-Cullin 1-F-box protein) protein complex, has been shown to mediate PHLPP1 degradation in tumours—as this regulation occurs via the PP2C domain conserved in both PHLPPs [38] , we tested PHLPP2-β-TrCP association in primary hepatocytes and hepatoma cells. Raptor overexpression markedly diminished proteosomal inhibitor-exposed PHLPP2-β-TrCP association ( Fig. 3i and Supplementary Fig. 6j ). Importantly, PHLPP1 levels or its association with β-TrCP was not altered ( Fig. 3d ), suggesting the specificity of free Raptor’s protection of PHLPP2 from β-TrCP-mediated proteosomal degradation. Hepatic PHLPP2 levels decline with aging and in obesity Free Raptor levels decline with aging and obesity—consistently, despite unchanged hepatic Phlpp2 gene expression ( Fig. 4a ), we observed lower PHLPP2 protein levels with aging and in dietary or genetic models of obesity ( Fig. 4b–d ). To test whether reduction in hepatic PHLPP2 is sufficient to induce steatosis, we constructed adenoviruses encoding shRNA targeting either Phlpp1 (Ad-shPHLPP1) or Phlpp2 (Ad-shPHLPP2). In primary hepatocytes, knockdown of PHLPP2 but not PHLPP1 increased Akt Ser473 phosphorylation ( Supplementary Fig. 7a ). Correspondingly, mice transduced with Ad-shPHLPP2 showed increased liver weight and hepatic steatosis ( Supplementary Fig. 7b,c ), mirroring the phenotype of mice transduced with constitutively active Akt (Ad-myrAkt) [39] , [40] . We next performed the converse experiment, to test whether adenoviral rescue of PHLPP2 (Ad-PHLPP2) in DIO mice would inhibit hepatic lipid accumulation. As expected, Ad-PHLPP2 mice showed decreased Akt Ser473 phosphorylation ( Fig. 4e ). In addition, despite unchanged body weight and adiposity ( Supplementary Fig. 8a,b ), Ad-PHLPP2 mice showed decreased liver weight ( Supplementary Fig. 8c ) and a trend towards lower hepatic triglyceride ( Fig. 4f ) and lipogenic gene expression ( Fig. 4g ), with an accompanying decrease in plasma triglyceride ( Fig. 4h ). 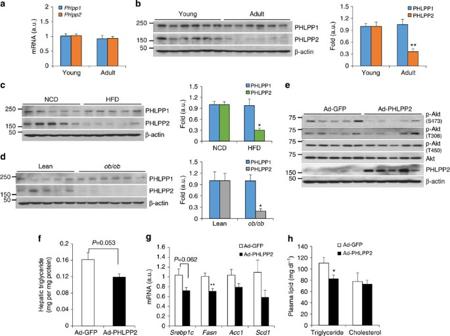Figure 4: Rescue of lower PHLPP2 in aging or obesity reduces lipogenesis. (a) Liver mRNA expression from young and adult mice (n=6 per each group). (b–d) Western blot from livers of young and adult (b), chow- and HFD-fed (c), or lean andob/ob(d) mice, normalized to β-actin. (e–h) Western blots from liver (e), hepatic triglyceride (f), liver lipogenic gene expression (g) and plasma lipids (h) in adult, HFD-fed Ad-GFP or Ad-PHLPP2 mice (n=6–7/group). *P<0.05, **P<0.01 as compared with the indicated control by two-way analysis of variance. All data are shown as the means±s.e.m. Figure 4: Rescue of lower PHLPP2 in aging or obesity reduces lipogenesis. ( a ) Liver mRNA expression from young and adult mice ( n =6 per each group). ( b – d ) Western blot from livers of young and adult ( b ), chow- and HFD-fed ( c ), or lean and ob/ob ( d ) mice, normalized to β-actin. ( e – h ) Western blots from liver ( e ), hepatic triglyceride ( f ), liver lipogenic gene expression ( g ) and plasma lipids ( h ) in adult, HFD-fed Ad-GFP or Ad-PHLPP2 mice ( n =6–7/group). * P <0.05, ** P <0.01 as compared with the indicated control by two-way analysis of variance. All data are shown as the means±s.e.m. Full size image These data suggest that preservation of free Raptor, via PHLPP2, can prevent hepatic steatosis, but to prove this, we co-transduced Ad-Raptor (or Ad-GFP control) mice with Ad-shControl, Ad-shPHLPP1 or Ad-shPHLPP2 adenoviruses. PHLPP2 knockdown restored Akt Ser473 phosphorylation in Ad-Raptor mice ( Fig. 5a ), resulting in hepatic and plasma triglyceride levels comparable to control mice ( Fig. 5b,c ), without altering body weight/adiposity or other serum metabolites ( Supplementary Fig. 9a–d ). PHLPP2 knockdown restored lipogenic gene expression ( Fig. 5d ), without affecting canonical mTORC1/2 signalling or activity ( Supplementary Fig. 9e ). Interestingly, Ad-myrAkt transduction in Ad-Raptor mice similarly increased liver triglyceride ( Fig. 5e ), buttressing our conclusion that free Raptor maintains normal hepatic lipogenesis/triglyceride content by increasing PHLPP2, to restrict Akt activation. 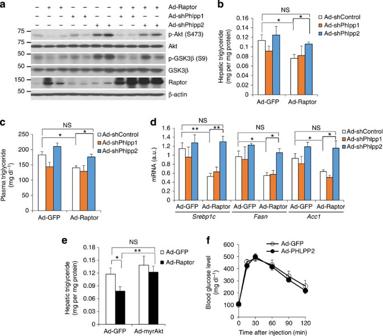Figure 5: Reduced liver triglyceride (TG) by free Raptor is PHLPP2-dependent. (a–d) Western blots from liver (a), hepatic TG (b), plasma TG (c) and liver lipogenic gene expression (d) of adult Ad-GFP and Ad-Raptor mice co-transduced with control (Ad-shControl), Ad-shPHLPP1 or Ad-shPHLPP2 adenoviruses, killed after a 16 h fast followed by 4 h refeeding (n=6 per group). (e) Hepatic TG from liver of adult Ad-GFP and Ad-Raptor mice co-transduced with control (GFP) or myrAkt adenovirus, killed after a 16 h fast followed by 4 h refeeding (n=6 per group). (f) GTT in adult, HFD-fed Ad-GFP or Ad-PHLPP2 mice (n=6–7 per group). *P<0.05, **P<0.01 as compared with the indicated control by two-way analysis of variance. All data are shown as the means±s.e.m. All blots are representative of three independent experiments, and samples within each group chosen randomly. Figure 5: Reduced liver triglyceride (TG) by free Raptor is PHLPP2-dependent. ( a – d ) Western blots from liver ( a ), hepatic TG ( b ), plasma TG ( c ) and liver lipogenic gene expression ( d ) of adult Ad-GFP and Ad-Raptor mice co-transduced with control (Ad-shControl), Ad-shPHLPP1 or Ad-shPHLPP2 adenoviruses, killed after a 16 h fast followed by 4 h refeeding ( n =6 per group). ( e ) Hepatic TG from liver of adult Ad-GFP and Ad-Raptor mice co-transduced with control (GFP) or myrAkt adenovirus, killed after a 16 h fast followed by 4 h refeeding ( n =6 per group). ( f ) GTT in adult, HFD-fed Ad-GFP or Ad-PHLPP2 mice ( n =6–7 per group). * P <0.05, ** P <0.01 as compared with the indicated control by two-way analysis of variance. All data are shown as the means±s.e.m. All blots are representative of three independent experiments, and samples within each group chosen randomly. Full size image Reduced hepatic Akt activity is typically associated with hyperglycaemia [41] . Surprisingly, but consistent with the phenotype of Ad-Raptor mice ( Supplementary Fig. 10a–c ), Ad-PHLPP2 mice showed normal glucose tolerance ( Fig. 5f ) and similar glucose and insulin levels as compared with control mice ( Supplementary Fig. 10d,e ). These data suggest that free Raptor, via PHLPP2, selectively regulates Akt’s effects on lipogenesis, while leaving intact Akt repression of hepatic glucose production. Although mTOR and Raptor expression tends to be tightly linked [24] , the association between these catalytic and primary scaffolding subunits of the mTORC1 complex is far more dynamic. Elegant biochemistry has shown that amino acid deprivation tightens, while rapamycin treatment loosens but does not break the mTOR–Raptor interaction [24] , [32] . While in vitro studies have hinted of the presence of an mTORC1-independent Raptor species [27] , [42] , our data proves for the first time the existence, and modulation by pathophysiologic (aging, obesity) stimuli, of free Raptor. Further study is required to determine whether free Raptor exists due to failure in association or true dissociation from mTOR, and whether the free and mTORC1-bound Raptor pools may interchange. In addition, what upstream signals (for example, alternative protein–protein interaction or a, post-translational modification on Raptor or another mTORC1 complex member) govern these event(s), and whether free Raptor affects other cellular processes are important questions that our lab is actively pursuing. Nevertheless, this first report of mTORC1-independent Raptor function suggests that its heretofore accepted role as a simple scaffold for mTOR catalytic activity is an oversimplification, and should prompt re-examination of the phenotypes of tissue-specific Raptor knockout mice. The Raptor/PHLPP2 axis provides yet another mechanism of interplay, albeit indirect, between the insulin/Akt and nutrient/mTOR pathways [9] , [21] , [37] . While there are likely additional determinants of hepatic PHLPP2, as evidenced by residual levels in L-Raptor livers, we postulate that insulin-Akt signalling, via free Raptor, may be responsible for its own regulation by PHLPP2. In fact, several predicted Akt and GSK3β phosphorylation sites exist in the C terminus of PHLPP2 within a β-TrCP-mediated destruction motif (phosphodegron), suggesting an Akt-dependent negative feedback loop to determine post-translational PHLPP2 stability to regulate Akt activity in obese liver. Conversely, a modest free Raptor-induced increase in PHLPP2 levels can reduce Akt-regulated DNL via increased Insig2a expression, but remarkably, does not impair glucose homoeostasis. This is striking contrast to the phenotype of hepatic mTORC2-deficient (and thus Akt Ser473 phosphorylation-incompetent) L-Rictor mice [21] , which fail to maximally activate Akt, leading to unchecked hepatic glucose output and glucose intolerance, closely approximating ‘complete’ hepatic insulin resistance [43] , [44] . Integrating these data, we propose a new model of insulin action ( Fig. 6 ) whereby Akt must be appropriately stimulated, but also inactivated by PHLPP2 in a timely fashion, to maintain normal hepatic physiology. Our model is consistent with the ‘bifurcation’ model of insulin signalling proposed by Brown & Goldstein [13] , and others [17] , but differs in the kinetics of events—inhibition of FoxO1 to repress gluconeogenesis is an ‘early’ event and requires the full force of Akt action [45] , but an extension of Akt activity by maintained Ser473 phosphorylation induces the ‘late’ lipogenic response by mTORC1-dependent [13] and -independent [9] pathways. 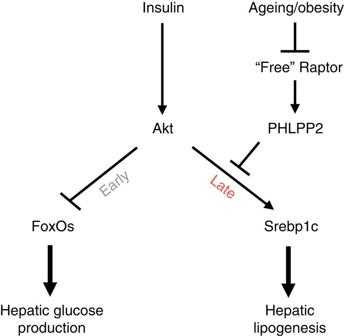Figure 6: A proposed model of free Raptor-mediated regulation of hepatic lipogenesis. Akt represents the common molecular hub of insulin regulation of hepatic glucose production and lipogenesis. In the post-prandial state, Akt-mediated FoxO nuclear exclusion occurs rapidly, after which Akt is dephosphorylated by PHLPP2 at Ser473 to terminate insulin action. In aging or obesity, loss of free Raptor destabilizes PHLPP2, leading to prolonged Akt activity and Srebp1c-dependent lipogenesis. Figure 6: A proposed model of free Raptor-mediated regulation of hepatic lipogenesis. Akt represents the common molecular hub of insulin regulation of hepatic glucose production and lipogenesis. In the post-prandial state, Akt-mediated FoxO nuclear exclusion occurs rapidly, after which Akt is dephosphorylated by PHLPP2 at Ser473 to terminate insulin action. In aging or obesity, loss of free Raptor destabilizes PHLPP2, leading to prolonged Akt activity and Srebp1c-dependent lipogenesis. Full size image PHLPPs have been the subject of considerable research in recent years, due to their therapeutic potential in neoplastic disease. Loss-of-heterozygosity has been observed at both PHLPP loci in multiple solid tumours [46] and a common PHLPP2 loss-of-function variant shown to reduce Akt dephosphorylation [47] has been observed in high-grade breast cancers. In combination with the known oncogenic role of Akt, these findings suggest that PHLPPs may have tumour suppressor activity. Enthusiasm for pharmacologic PHLPP activators, such as HDAC3 inhibitors [48] or adenylate cyclase activators [49] , has been tempered by speculated interference with normal Akt function and potential to cause new-onset T2D [46] , consistent with epidemiologic studies showing increased PHLPP1 , but importantly not PHLPP2 , expression in adipose or muscle of obese/T2D [50] , [51] . Our, gain- and loss-of-function studies show that PHLPP1 has little function in liver, whereas hepatic PHLPP2 levels/activity dissociate Akt functions in liver to reduce lipogenesis without adversely affecting glucose tolerance. Our data would suggest that application of putative PHLPP2 agonists or liver-specific delivery of non-specific PHLPP activators [52] have the potential to stem the tide of obesity-induced NAFLD. Experimental animals 8-week-old male wild-type C57/BL/6 mice fed on standard chow or HFD were purchased from Jackson Labs. We injected AAV8-TBG-GFP or AAV8-TBG-Cre (Penn Vector Core) into male Raptor flox/flox (Jackson Laboratory; stock number 013188) mice fed on standard chow or HFD, and characterized the mice at 2 weeks after AAV injection. Number of animals used in experiments was chosen to ensure adequate power to detect experimental difference with alpha set to 0.05. All animal experiments were conducted in accordance with guidelines of, and were explicitly approved by, the Columbia University Institutional Animal Care and Use Committee. Metabolic analyses Blood glucose (blood taken from tail vein) was measured using a glucometer (OneTouch) and plasma insulin concentrations were measured using a mouse insulin ELISA kit (Mercodia). Glucose tolerance tests were performed by intraperitoneal injection of 2 g per kg body weight glucose after a 16 h fast. Hepatic lipids were extracted by the Folch method [53] , and plasma and hepatic triglyceride, Cholesterol E and non-esterified fatty acid were measured using a colorimetric assay from Thermo or Wako Chemicals, according to the manufacturer’s protocol. We measured hepatic DNL by measuring the amount of newly synthesized fatty acid present in the liver 1 h after intraperitoneal injection of 1mCi of 3 H 2 O (ref. 54 ). Gel filtration chromatography and crosslinking assay Liver tissues from three independent mice were pooled and lysed in hypotonic buffer (40 mM Tris-HCl (pH 7.5)) [42] including protease inhibitors (Pierce) by repeated passage with a 27-gauge needle. The lysates were centrifuged at 14,000 r.p.m. for 15 min, and the supernatants were further centrifuged. The supernatant fraction was filtered with a PVDF membrane and then applied to a Superose 6 column (Amersham Biosciences) and eluted with 40 mM Tris-HCl (pH 7.5) and 150 mM NaCl. The column was calibrated with the Gel Filtration Marker Kit (Sigma). Liver tissues were lysed in 1% Triton X-100 lysis buffer [24] including protease and phosphatase inhibitors with or without 2.5 mg ml −1 dithiobis[succinimidylpropionate] or disuccinimidyl suberate (Pierce), and incubated for 2 h on ice. Crosslinking reactions were quenched by adding 1 M Tris-HCl (pH 7.5) followed by an additional 30 min incubation. For in vivo crosslinking assays, dithiobis[succinimidylpropionate] or disuccinimidyl suberate were added to a final concentration in the cell culture medium of 1 mg ml −1 and reactions quenched by adding Tris-HCl (pH 7.5). Equal protein amounts were then analysed by either immunoprecipitation or immunoblotting directly. Adenovirus studies The GFP, Raptor and PHLPP1/2 adenoviruses have been described [23] , [55] . The HA-Flag-PHLPP2 adenovirus was constructed by inserting a Flag sequence into HA-PHLPP2 vector (Addgene #22403, courtesy of Alexandra Newton) and adenoviruses encoding HA-Flag-PHLPP2 generated by Welgen, Inc. (Worcester, MA). Mouse shPhlpp1 or 2 target sequences were selected among three candidate sequences, respectively, and adenoviruses encoding shPhlpp1 or 2 generated by Welgen, Inc. Adenovirus expressing shmTOR, shRaptor and shRictor was generated by homologous recombination between pAd-Easy1 and pAd-Track vector. For in vivo studies, we injected 5 × 10 8 or 2.5 × 10 8 purified viral particles per gram body weight; we performed metabolic analysis on days 3–5 and killed the mice at day 8 or 10 after injection. Infection with adenovirus in primary hepatocytes or Hepa1c1c7 cells was performed at 2.5, 5, or 10 multiplicity of infection. Primary hepatocyte cultures Primary mouse hepatocytes were isolated as previously described [56] —in brief, mice were anaesthetized with a ketamine/xylazine mixture (Sigma), abdominal cavity exposed and inferior vena cava catheterized with a 23-gauge catheter (Becton Dickinson). The superior vena cava was clamped, portal vein was transected and Hepes-based perfusion solution infused into the liver for 2 min at 5 cc min −1 followed by type I collagenase (Worthington Biochemicals), including protease inhibitor caplets (Boehringer Mannheim), for 18 min at the same flow rate. Liver cells were filtered, mixed with Percoll and spun at 100 g to remove dead cells and non-hepatocytes. After two washes, cells were plated at 0.8 × 10 6 cells per well of six-well dish in Williams E supplemented with 5% FCS (Invitrogen). For inhibitor experiments, we treated hepatocytes with 20 nM rapamycin (Cell Signaling), 250 nM Torin1 or vehicle for either 1 or 24 h. The construct expressing HA/Ub was transfected using Lipofectamine 3000 (Invitrogen) according to the manufacture’s recommendation. Western blotting and co-immunoprecipitation Liver tissues or cells were lysed in a Triton-based or 0.3% CHAPS lysis buffer [24] and whole-cell lysates were obtained by subsequent centrifugation. Immunoblots were conducted on 3–5 samples randomly chosen within each experimental cohort with antibodies against Raptor (#2280), Akt (#9272), p-Akt (S473, #4060), p-Akt (T308, #9275), p-Akt1 (S473, #9018), p-Akt2 (S474, #8599), p-Akt (T450, #12178), p-Akt substrate (#9614), PKCα (#2056), p-GSK3β (S9, #9336), GSK3β (#9315) mTOR (#2983), Rictor (#2140), GβL (#3274), p-S6 (S240/244, #2215), S6 (#2217), p-4E-BP1 (T37/46, #2855), β-TrCP (#4394), p-IRS1 (S636/639, #2388) and β-actin (#4970) from Cell Signaling; mTOR (sc-1549) and α-tubulin (sc-12462) from SantaCruz Biotechnology, Inc.; PHLPP1 (A300-660A) and PHLPP2 (A300-661A) from Bethyl Laboratories, Inc.; a polyclonal antibody against Raptor (#42-4,000) from Invitrogen; as well as Protein A-HRP (10-1,023) from Pierce. Primary antibodies were used at a 1:1,000 dilution. Uncropped images for all western blots can be found in Supplementary Fig. 11 . For co-immunoprecipitation assays, liver extracts or cells were mixed with anti-mTOR or PHLPP2 antibody immobilized on Protein A or G-Sepharose (Invitrogen). Quantitative reverse transcription PCR We isolated RNA with TRIzol (Invitrogen) or an RNeasy Mini kit (Qiagen), synthesized complementary DNA with High-Capacity cDNA Reverse Transcription kit (Applied Biosystems) and performed quantitative reverse transcription PCR with a GoTaq SYBR Green qPCR kit (Promega) in a CFX96 Real-Time PCR detection system (Bio-Rad). Primer sequences are available in Supplementary Table 1 . In vitro mTORC1 or Akt kinase assay Liver lysates were immunoprecipitated with anti-mTOR or anti-Akt antibody (sepharose bead conjugated) and the immunoprecipitates were incubated with 4E-BP1 or GSK3 fusion protein substrate in kinase buffer for 30 min at 30 °C. Reactions were terminated by SDS loading buffer. The samples were separated on SDS–PAGE, and the p-4E-BP1 (T37/46) or p-GSK3β (S9) was detected by immunoblot. Statistical analysis We performed comparisons using two-way analysis of variance. All data are shown as the means±s.e.m. How to cite this article: Kim, K. et al. mTORC1-independent Raptor prevents hepatic steatosis by stabilizing PHLPP2. Nat. Commun. 7:10255 doi: 10.1038/ncomms10255 (2016).